Selective C-H trifluoromethoxylation of (hetero)arenes as limiting reagent Methods for direct C-H trifluoromethoxylation of arenes and heteroarenes are rare, despite the importance of trifluoromethoxylated compounds for pharmaceuticals, agrochemicals, and material sciences. Especially selective C-H trifluoromethoxylation of pyridines remains a formidable challenge. Here we show a general late-stage C-H trifluoromethoxylation of arenes and heteroarenes as limiting reagent with trifluoromethoxide anion. The reaction is mediated by silver salts under mild reaction conditions, exhibiting broad substrate scope and wide functional-group compatibility. In addition, ortho -position selective C-H trifluoromethoxylation of pyridines is observed. The method is not only applicable to the gram-scale synthesis of trifluoromethoxylated products but also allows efficient late-stage C-H trifluoromethoxylation of marketed small-molecule drugs, common pharmacophores and natural products. Trifluoromethoxy (OCF 3 ) groups are becoming increasingly important in pharmaceuticals, agrochemicals, and material sciences. In particular, the introduction of trifluoromethoxy groups into arenes and heteroarenes is of paramount importance in organic molecules because of their outstanding electronegativity and high lipophilicity (Fig. 1a ) [1] , [2] , [3] . For example, Riluzole is the first approved drug for the treatment of patients with neurological diseases such as amyotrophic lateral sclerosis [4] ; Celikalim is a potent potassium channel opener in human airway smooth muscles [5] . Many pesticides also contain the OCF 3 group, such as Triflumuron, Indoxacarb, and Thifluzamide [6] . In addition, 2-(trifluoromethoxy)pyridine and 2-(trifluoromethoxy)quinoline derivatives are especially useful for drugs and agrochemicals [7] . Despite the development of methods for the synthesis of trifluoromethoxylated compounds that has been an area of great interest, only a few examples have been reported for the synthesis of trifluoromethoxylated arenes and heteroarenes [8] , [9] , [10] , [11] , [12] , [13] . Especially the most atom economical C-H trifluoromethoxylation of arenes and heteroarenes remains a formidable challenge due to the reversible decomposition of trifluoromethoxide anion and the limited number of available trifluoromethoxylation reagents [14] , [15] , [16] , [17] , [18] , [19] , [20] , [21] , [22] , [23] , [24] , [25] , [26] , [27] , [28] , [29] , [30] , [31] , [32] . Traditional methods for the synthesis of aryl trifluoromethyl ethers employed classical approaches such as reactions of phenols via fluoroformate or chlorothionoformate intermediates, followed by nucleophilic fluorination with antimony trifluoride, hydrofluoric acid, or sulfur tetrafluoride at 100–160 °C [33] , [34] , [35] , [36] , [37] . The harsh reaction conditions can only be tolerated by structurally simple phenol derivatives. In this context, Togni reported the successful trifluoromethylation of 2,4,6-trimethylphenol with the Togni’s reagent and up to 15% yield of the desired aryl trifluoromethyl ether [38] , while Wu reported the synthesis of N -heteroaromatic trifluoromethoxy compounds by direct O-CF 3 bond formation with the Togni’s reagent [39] . Umemoto reported the trifluoromethylation of phenols using Umemoto’s reagent under photoirradiation at −100 °C [40] . In 2014, Ngai reported a two-step sequence of O -trifluoromethylation of N -aryl- N -hydroxylamine and intramolecular OCF 3 migration to prepare trifluoromethoxylated aniline derivatives [41] , [42] . Qing reported a silver-mediated oxidative trifluoromethylation of phenols with Ruppert–Prakash reagent [43] . Both of these reactions were realized with CF 3 reagents (Fig. 1b ). Recently, Ritter reported a silver-mediated cross-coupling of aryl stannanes and aryl boronic acids to produce trifluoromethoxylated arenes with tris(dimethylamino)sulfonium trifluoromethoxide [44] . The trifluoromethoxylation of arenediazonium tetrafluoroborates with stoichiometric silver or stoichiometric copper was described by Tang and our group [45] , [46] . The synthesis of phenyl and naphthyl trifluoromethyl ether was reported by the groups of Kolomeitsev and Hu, via the addition of trifluoromethoxide to benzyne and α-naphthyne generated in situ [47] , [48] . Hartwig reported the trifluoromethoxylation of quinoline and phenanthridine N -oxide to synthesize heteroaromatic trifluoromethyl ethers [49] . These reactions utilized pre-functionalized arenes and heterocyclic N -oxide as substrates, which might hamper the applicability for late-stage modifications of complex small molecules (Fig. 1c ). Fig. 1: Arene and heteroarene C-H trifluoromethoxylation. a Applications of OCF 3 -containing compounds. b Trifluoromethylation with [CF 3 ]. c Trifluoromethoxylation with anionic OCF 3 . d Trifluoromethoxylation with OCF 3 radical. e Direct C-H trifluoromethoxylation with anionic OCF 3 . Full size image Direct functionalization of a C-H bond with a trifluoromethoxy group would be advantageous for the step-economic synthesis of trifluoromethoxy ethers. However, only a few examples of direct C-H trifluoromethoxylation of (hetero)arenes were reported to date. In 2018, the groups of Ngai and Togni independently reported the intermolecular C-H trifluoromethoxylation of (hetero)arenes employing a photoredox catalyst with the N -OCF 3 reagents [50] , [51] , [52] . Mechanism involving a OCF 3 radical was proposed. However, excess of (hetero)arenes was required to achieve good yields of the desired products as mixture of isomers ( o : m : p ). In addition, no example of ortho -position selective C-H trifluoromethoxylation of pyridines was reported (Fig. 1d ). It is certainly highly desirable to develop an efficient and general approach for the selective (hetero)aromatic C-H trifluoromethoxylation, preferably with 1 equivalent of (hetero)arenes, which would be a powerful tool for late-stage trifluoromethoxylation of drug candidates, agrochemicals, and natural products. Herein we report a silver-mediated direct C-H trifluoromethoxylation with arenes and heteroarenes as the limiting reagent (Fig. 1e ). Compared to previous reports, exclusive ortho -selective C-H trifluoromethoxylation of pyridines and selective C-H trifluoromethoxylation of ortho - and para -position of arenes are achieved. This method not only exhibits high efficiency and wide functional-group compatibility but also allows the late-stage trifluoromethoxylation of bioactive molecules and natural product derivatives. Investigations of reaction conditions and scope In order to improve the regioselectivity of the direct (hetero)aromatic C-H trifluoromethoxylation reactions, we envisioned to in situ generate the proposed Ag(II)OCF 3 intermediate in the presence of silver salts, oxidant, and trifluoromethyl arylsulfonate (TFMS), which was triggered by fluoride ions to deliver OCF 3 anion as reported in our previous results [53] , [54] , [55] . The Ag(II)OCF 3 intermediate could coordinate with pyridine substrates and give the desired products through the trifluoromethoxylation at the ortho -position of pyridines. 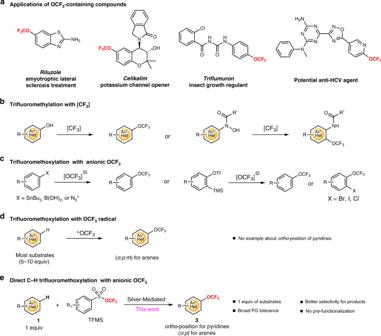Fig. 1: Arene and heteroarene C-H trifluoromethoxylation. aApplications of OCF3-containing compounds.bTrifluoromethylation with [CF3].cTrifluoromethoxylation with anionic OCF3.dTrifluoromethoxylation with OCF3radical.eDirect C-H trifluoromethoxylation with anionic OCF3. In order to test our hypothesis, we chose 4-( tert -butyl)pyridine 1a as the model substrate for the direct trifluoromethoxylation of C(sp 2 )-H bonds (Table 1 ). No desired product 3a was observed in the absence of silver salts (Table 1 , entry 1). We were delighted to find that 62% yield of the desired product 3a was observed when AgF 2 was used as the silver salts (Table 1 , entries 2–6). The oxidant was important for this transformation, and Selectfluor could give the best yield. Switching to other oxidants, Selectfluor II, N -fluorobenzenesulfonimide, PhI(OAc) 2 , and K 2 S 2 O 8 could generate 3a in lower yields (Table 1 , entries 7–10). In addition, CsF was the best fluoride source, which reacted with TFMS to generate CsOCF 3 . The poorly soluble CsOCF 3 ensured that the intermediate Ag(II)OCF 3 was generated gradually, which might slow down the decomposition of OCF 3 anion. Less than 10% yields of the desired products were detected in control experiments with no CsF or oxidant. It was worth mentioning that exclusive selective for C-H trifluoromethoxylation adjacent to nitrogen was observed. The main by-product was 4-( tert -butyl)−2-fluoropyridine, which was generated from fluorination of pyridines with AgF 2 . After extensive screening of various solvents, different substitutions on TFMS, and temperatures (see more details in Supplementary Tables 1 – 8 ), the ideal conditions under 1.0 equiv of AgF 2 , 2.0 equiv of Selectfluor, 3.0 equiv of CsF, 3.0 equiv of TFMS ( 2 ) in dimethyl carbonate (DMC) under N 2 atmosphere at 35 °C were found to produce the highest yields of the desired product 3a (method A). Table 1 Optimization of reaction conditions a . Full size table With the optimized reaction conditions in hand, this method was further applied to a number of pyridines with representative electron-rich substitutions, providing the corresponding ortho -selective C-H trifluoromethoxylation products in good yields (Fig. 2 ). However, the extension of the method to the trifluoromethoxylation of pyridines with electron-deficient substitution resulted in relatively low efficiency, and there were a lot of starting material recovered. This might be attributed to that Selectfluor ( E 1/2 red = +0.33 V vs saturated calomel electrode (SCE) in CH 3 CN) is not strong enough to oxidize electron-deficient substrates well [56] . We then switched Selectfluor to AgF 2 (the redox potential of the Ag(I)/Ag(II) couple is +1.98 V vs SCE) [57] , a stronger oxidant and powerful reagent in C-H fluorination of pyridines with either electron-donating or electron-withdrawing substituents [58] , [59] , [60] , [61] , [62] . Gratifyingly, the expected trifluoromethoxylation products could be achieved in high efficiency when the reaction was carried out with AgF 2 (4.0 equiv) as the oxidant and fluoride source in MeCN solution at 10 °C (method B). The generality of the method was then clearly demonstrated by the synthesis of trifluoromethoxylated products (3g, 3j, 3k, 3m, 3p to 3t) in satisfactory yields from the corresponding electron-deficient pyridines (Fig. 2 ). In contrast, the extension of method B to the trifluoromethoxylation of electron-rich pyridines resulted in low yields with the generation of large amounts of fluorinated by-products. Perhaps, before the Ag(II)OCF 3 intermediate was formed, AgF 2 reacted with electron-rich pyridines under this condition to give the fluorinated by-products. Fig. 2: Substrate scope of simple arenes and heteroarenes. a Method A: 1 (1.0 equiv), AgF 2 (1.0 equiv), TFMS ( 2 ) (3.0 equiv), Selectfluor (2.0 equiv), CsF (3.0 equiv), DMC, N 2 , 35 °C. b Method B: 1 (1.0 equiv), AgF 2 (4.0 equiv), TFMS ( 2 ) (4.0 equiv), MeCN, N 2 , 10 °C. c Method C: 1 (1.0 equiv), AgF 2 (1.0 equiv), TFMS ( 2 ) (4.0 equiv), Selectfluor (2.0 equiv), CsF (4.0 equiv), 4- tert -butyl-2,6-bis(4- tert -butylpyridin-2-yl)pyridine (0.1 equiv). DMC, N 2 , 35 °C. d Method D: 1 (1.0 equiv), AgF 2 (4.0 equiv), TFMS ( 2 ) (4.0 equiv), di(pyridin-2-yl)methanone (0.1 equiv), MeCN, N 2 , 10 °C. e K 2 S 2 O 8 was used instead of Selectfluor. f Yields were determined by the 19 F NMR spectrum using benzotrifluoride as internal standards. Full size image Having established the reaction protocol for the C( sp 2 )-H trifluoromethoxylation of pyridines, we next focused on the C( sp 2 )-H trifluoromethoxylation of arenes and other heterocyclic compounds, which are certainly of high value. Direct application of the method A to the trifluoromethoxylation of model substrate 2-chloro-6-methoxyquinoline ( 1ff ) resulted in a low conversion (5% yield). This phenomenon might be ascribed to the relatively low concentration and stability of Ag(II)–OCF 3 species responsible for trifluoromethoxylation. A possible solution was adding a ligand to coordinate with Ag(II)–OCF 3 species like pyridine, which could increase the solubility and stability of intermediate. We then screened a number of ligands based on method A. With a catalytic amount of 4,4′,4″-tri- tert -butyl-2,2′:6′,2″-terpyridine as the ligand, the yield of the trifluoromethoxylation reaction was increased from 5% to 76% (see Supplementary Table 9 ). The optimal conditions were thus determined as to run the reaction in DMC at 35 °C with AgF 2 (1 equiv) as the reaction medium, Selectfluor (2 equiv) as the oxidant, TFMS (4 equiv) as the OCF 3 source, CsF (4 equiv) as the fluorine source, and 4,4′,4″-tri- tert -butyl-2,2′:6′,2″-terpyridine (0.1 equiv) as the ligand (method C). Method C was then applied to the trifluoromethoxylation of a variety of (hetero)arenes, and the results are summarized in Fig. 2 . Substrates with electron-donating substituents on the (hetero)aromatic ring all underwent C-H trifluoromethoxylation smoothly, furnishing the corresponding products in satisfactory yields. However, the same problem appeared in the relatively electron-deficient substrates, which need AgF 2 (4 equiv) as the oxidant and di(pyridin-2-yl)methanone (0.1 equiv) as the ligand (method D). In addition, <5% yield of trifluoromethoxylated products with more electron-deficient substrates, such as (trifluoromethyl)benzene and nitrobenzene, were observed even with method D, and 11% yield was obtained when benzene was used as the substrate. Although this trifluoromethoxylation method was not suitable for electron-deficient arenes, mono-, di-, and tri-substituted pyridines with both electron-donating and electron-withdrawing groups are tolerated, and other heteroaromatic substrates, such as quinoline, indole, thiophene, chromone, and coumarin, were also successfully employed to provide the corresponding trifluoromethoxylated products ( 3ee – 3jj ). A good range of functional groups including ester, ether, ketone, acetal, nitrile, nitro, hydroxyl, and halogens were well tolerated under these mild reaction conditions. Compared to the previous reports, only 1 equiv of (hetero)arenes was used in the reaction, and exclusive ortho -position selective C-H trifluoromethoxylation of pyridines was achieved. In addition, compounds 3p and 3ff were prepared in a gram scale in 75% and 73% isolated yield, respectively, which demonstrates the scalability of this method. The direct trifluoromethoxylation of aromatic C-H bonds could facilitate access to trifluoromethoxylated derivatives of complex small molecules that would otherwise be difficult to produce. Given that a trifluoromethoxy group is present in a range of small-molecule drugs and preclinical candidates, we examined a number of well-known natural products or drug derivatives (Fig. 3 ). Each of these architecturally complex molecules underwent (hetero)aryl C-H trifluoromethoxylation to achieve the corresponding trifluoromethoxylated products in moderate yields ( 4kk – 4tt , 22–76% yield). For example, etoricoxib, a selective cyclooxygenase-2 inhibitor and a non-steroidal anti-inflammatory drug, was used as the substrate to give the corresponding trifluoromethoxylated product 4kk in 22% yield via method B. The trifluoromethoxylation of tropicamide, an anticholinergic drug containing a unprotected hydroxyl group and an acidic α-phenyl amide, proceeded with method A to form the product 2ll . 3-(Pyridin-4-yloxy)propyl ester of β-lactamase inhibitor sulbactam underwent ortho -position selective C-H trifluoromethoxylation of the pyridine ring to produce 4oo in 40% isolated yield. In another case, Tanshinone IIA with significant effect in treating coronary heart disease was nicely converted to its trifluoromethoxylated product 4rr in 32% yield via method C. The trifluoromethoxylation reaction of apigenin derivative, which is a natural product found in many plants, proceeded smoothly to provide the corresponding product ( 4ss ) in 76% yield. Finally, a trifluoromethoxylated derivative of hypolipidemic drug fenofibrate was readily prepared in 35% yield via method D. The structure of the products 4kk and 4ss were confirmed by X-ray crystallographic analysis. These results illustrated the ability to conduct the late-stage (hetero)aromatic C-H trifluoromethoxylation of complex structures. Fig. 3: Late-stage C-H trifluoromethoxylation of natural products and drug derivatives. a Method A: 1 (1.0 equiv), AgF 2 (1.0 equiv), TFMS ( 2 ) (3.0 equiv), Selectfluor (2.0 equiv), CsF (3.0 equiv), DMC, N 2 , 35 °C. b Method B: 1 (1.0 equiv), AgF 2 (4.0 equiv), TFMS ( 2 ) (4.0 equiv), MeCN, N 2 , 10 °C. c Method C: 1 (1.0 equiv), AgF 2 (1.0 equiv), TFMS ( 2 ) (4.0 equiv), Selectfluor (2.0 equiv), CsF (4.0 equiv), 4- tert -butyl-2,6-bis(4- tert -butylpyridin-2-yl)pyridine (0.1 equiv). DMC, N 2 , 35 °C. d Method D: 1 (1.0 equiv), AgF 2 (4.0 equiv), TFMS ( 2 ) (4.0 equiv), di(pyridin-2-yl)methanone (0.1 equiv), MeCN, N 2 , 10 °C. e K 2 S 2 O 8 was used instead of Selectfluor. Full size image Although the mechanistic details of this transformation are not clear, a series of experiments were performed to gain insight into the mechanism of the reactions (Fig. 4a ). No trifluoromethoxylated product 3h was observed when 2-fluoropyridine reacted with TFMS in the presence of the base. In all, 29% yield of trifluoromethoxylated product 3a and 19% yield of by-product 3a’ were observed when AgF 2 was replaced by AgOTf. These results indicated that the trifluoromethoxylated products were not generated from nucleophilic aromatic substitutions (S N Ar) of the 2-fluoropyridine [63] . When N -fluoropyridinium salt was used as the substrate, no desired product 3h was observed. Furthermore, kinetic isotopic effect experiments were conducted by treatment of pyridine and deuterated pyridine under the reaction conditions. A k H / k D value of 2.1 was obtained in a competitive reaction and 1.8 in parallel reactions on the basis of 19 F nuclear magnetic resonance analysis, which was indicative of a primary kinetic isotope effect. In addition, no trifluoromethoxylated product was formed when the radical inhibitor 2,2,6,6-tetramethyl-1-piperidinyloxy (1 equiv) or 2,6-di- tert -butyl-4-methylphenol (4 equiv) was added, and electron paramagnetic resonance experiments were performed with the addition of free radical spin trapping agent α-(4-pyridyl N -oxide)- N - tert -butylnitrone (POBN). The signals of unknown organic radicals were observed, which did not match the previously reported POBN-OCF 3 • adducts [51] (see more details in Supplementary Fig. 2 ). Furthermore, several pieces of data indicated that a free OCF 3 radical was not involved in the reaction. First, the exclusive selectivity for trifluoromethoxylation at the 2-position of pyridines was observed, which contrasts with the mixture of isomeric products formed in varying amounts for the addition of alkyl, aryl, and fluoroalkyl radicals to pyridines depending on the steric and electronic properties of the reactants [64] , [65] , [66] , [67] . Second, 2,6-dimethylpyridine did not undergo trifluoromethoxylation, while an OCF 3 radical should add to the 3- or 4-position. Third, C-H trifluoromethoxylation of tert -butylbenzene ( 3u ) could get ( o , p )-products, which was different from the previous report with ( o : m : p ) isomers via an OCF 3 radical by Ngai [52] , [68] . Finally, compared to the previous reports with moderate yields, <5% yield of trifluoromethoxylated products were observed using more electron-deficient arenes as the substrates in our reaction. Fig. 4: Mechanistic studies and proposed mechanism. a Mechanistic studies. b Proposed mechanism for pyridines. c Proposed mechanism for arenes. Full size image On the basis of these mechanistic investigations, we proposed the mechanism depicted in Fig. 4 . When pyridines were used as the substrates (Fig. 4b ), the mechanism would involve initial coordination of AgF 2 to pyridines, then reacted with TFMS to produce intermediate I , followed by single-electron transfer between Ag(II)OCF 3 and pyridines leads to the generation of intermediated II , followed by addition OCF 3 anion to get intermediate III , which is oxidized to form cation intermediate IV , then generated the desired products by proton abstraction. When arenes were the substrates (Fig. 4c ), the mechanism was similar to pyridines with the production of intermediate V first. 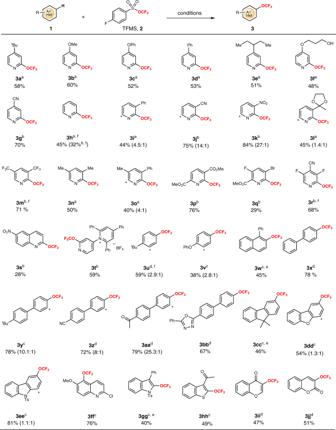Fig. 2: Substrate scope of simple arenes and heteroarenes. aMethod A: 1 (1.0 equiv), AgF2(1.0 equiv), TFMS (2) (3.0 equiv), Selectfluor (2.0 equiv), CsF (3.0 equiv), DMC, N2, 35 °C.bMethod B: 1 (1.0 equiv), AgF2(4.0 equiv), TFMS (2) (4.0 equiv), MeCN, N2, 10 °C.cMethod C: 1 (1.0 equiv), AgF2(1.0 equiv), TFMS (2) (4.0 equiv), Selectfluor (2.0 equiv), CsF (4.0 equiv), 4-tert-butyl-2,6-bis(4-tert-butylpyridin-2-yl)pyridine (0.1 equiv). DMC, N2, 35 °C.dMethod D: 1 (1.0 equiv), AgF2(4.0 equiv), TFMS (2) (4.0 equiv), di(pyridin-2-yl)methanone (0.1 equiv), MeCN, N2, 10 °C.eK2S2O8was used instead of Selectfluor.fYields were determined by the19F NMR spectrum using benzotrifluoride as internal standards. 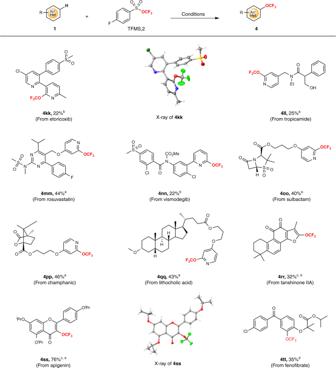Fig. 3: Late-stage C-H trifluoromethoxylation of natural products and drug derivatives. aMethod A: 1 (1.0 equiv), AgF2(1.0 equiv), TFMS (2) (3.0 equiv), Selectfluor (2.0 equiv), CsF (3.0 equiv), DMC, N2, 35 °C.bMethod B: 1 (1.0 equiv), AgF2(4.0 equiv), TFMS (2) (4.0 equiv), MeCN, N2, 10 °C.cMethod C: 1 (1.0 equiv), AgF2(1.0 equiv), TFMS (2) (4.0 equiv), Selectfluor (2.0 equiv), CsF (4.0 equiv), 4-tert-butyl-2,6-bis(4-tert-butylpyridin-2-yl)pyridine (0.1 equiv). DMC, N2, 35 °C.dMethod D: 1 (1.0 equiv), AgF2(4.0 equiv), TFMS (2) (4.0 equiv), di(pyridin-2-yl)methanone (0.1 equiv), MeCN, N2, 10 °C.eK2S2O8was used instead of Selectfluor. 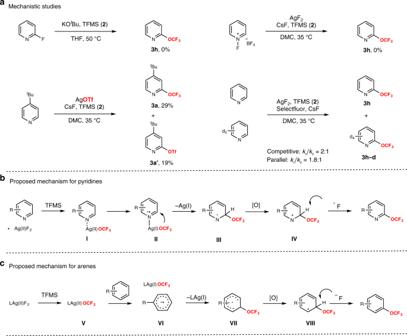Fig. 4: Mechanistic studies and proposed mechanism. aMechanistic studies.bProposed mechanism for pyridines.cProposed mechanism for arenes. The subsequent single-electron transfer between Ag(II)OCF 3 and arenes leads to the generation of Ag(I)OCF 3 species and intermediated VI , followed by addition OCF 3 anion to get intermediate VII , which is oxidized to form carbocation intermediate VIII , then generated the desired products by proton abstraction. In conclusion, we have presented a silver-mediated late-stage C-H trifluoromethoxylation reaction with arenes and heteroarenes as limiting reagent, which allows efficient late-stage trifluoromethoxylation of a variety of organic molecules and known drugs. Although the trifluoromethoxylation method reported herein needs stoichiometric amount silver salts, it affords exclusive ortho -position selective C-H trifluoromethoxylation of pyridines. The reaction is operationally simple under mild conditions, tolerates a large range of functional groups, and is applicable to the gram-scale synthesis of trifluoromethoxylated products. It is anticipated to serve for the late-stage modification to quickly obtain structural diversity in drug development. General procedure for the synthesis of trifluoromethoxylated products Method A: In a glove box, to a 15.0-mL sealed tube were added in sequence Selectfluor (354 mg, 1.00 mmol, 2.00 equiv), AgF 2 (72 mg, 0.50 mmol, 1.00 equiv), CsF (228 mg, 1.50 mmol, 3.00 equiv), 10.0 mL DMC, pyridines (0.50 mmol, 1.00 equiv), and TFMS (240 μL, 1.50 mmol, 3.00 equiv). The mixture was stirred at 35 °C for 24 h. After cooling to 23 °C, the reaction mixture was filtered through a short plug of silica gel eluting with approximately 25 mL of CH 2 Cl 2 or EtOAc. The filtrate was concentrated, and the residue was purified by chromatography on silica gel. Method B: In a glove box, to a 2.0-mL sealed tube were added in sequence pyridines (0.50 mmol, 1.00 equiv), 0.5 mL MeCN (the solvent was pre-cooled to −30 °C), and TFMS (320 μL, 2.00 mmol, 4.00 equiv), then AgF 2 (290 mg, 2.0 mmol, 4.00 equiv) was added at once in one portion. The mixture was stirred at 10 °C for 36 h. After warming up to 23 °C, the reaction mixture was filtered through a short plug of silica gel eluting with approximately 25 mL of CH 2 Cl 2 or EtOAc. The filtrate was concentrated, and the residue was purified by chromatography on silica gel. Method C: In a glove box, to a 15.0-mL sealed tube were added in sequence Selectfluor (354 mg, 1.0 mmol, 2.00 equiv) or K 2 S 2 O 8 (270 mg, 1.0 mmol, 2.00 equiv), AgF 2 (72 mg, 0.50 mmol, 1.00 equiv), CsF (304 mg, 2.00 mmol, 4.00 equiv), 4- tert -butyl-2,6-bis(4- tert -butylpyridin-2-yl)pyridine (20.0 mg, 0.05 mmol, 0.10 equiv), 10.0 mL DMC, arenes or heteroarenes (0.50 mmol, 1.00 equiv), and TFMS (320 μL, 2.00 mmol, 4.00 equiv). The mixture was stirred at 35 °C for 24 h. After cooling to 23 °C, the reaction mixture was filtered through a short plug of silica gel eluting with approximately 25 mL of CH 2 Cl 2 or EtOAc. The filtrate was concentrated, and the residue was purified by chromatography on silica gel. Method D: In a glove box, to a 2.0-mL sealed tube were added in sequence di(pyridin-2-yl)methanone (9.2 mg, 0.05 mmol, 0.10 equiv), AgF 2 (290 mg, 1.0 mmol, 4.00 equiv), 1.0 mL MeCN, arenes or heteroarenes (0.50 mmol, 1.00 equiv), and TFMS (320 μL, 2.00 mmol, 4.00 equiv). The mixture was stirred at 10 °C for 36 h. After warming up to 23 °C, the reaction mixture was filtered through a short plug of silica gel eluting with approximately 25 mL of CH 2 Cl 2 or EtOAc. The filtrate was concentrated, and the residue was purified by chromatography on silica gel.